Surface symmetry-breaking and strain effects on orbital occupancy in transition metal perovskite epitaxial films The electron occupancy of 3d-orbitals determines the properties of transition metal oxides. This can be achieved, for example, through thin-film heterostructure engineering of AB O 3 oxides, enabling emerging properties at interfaces. Interestingly, epitaxial strain may break the degeneracy of 3 d - e g and t 2 g orbitals, thus favoring a particular orbital filling with consequences for functional properties. Here we disclose the effects of symmetry breaking at free surfaces of AB O 3 perovskite epitaxial films and show that it can be combined with substrate-induced epitaxial strain to tailor at will the electron occupancy of in-plane and out-of-plane surface electronic orbitals. We use X-ray linear dichroism to monitor the relative contributions of surface, strain and atomic terminations to the occupancy of 3z 2 -r 2 and x 2 -y 2 orbitals in La 2/3 Sr 1/3 MnO 3 films. These findings open the possibility of an active tuning of surface electronic and magnetic properties as well as chemical properties (catalytic reactivity, wettability and so on). Electron filling of 3 d -orbitals of transition metal oxides plays a crucial role regarding their properties. Indeed, tailoring their electron occupancy and their relative orientation in crystal lattices has allowed disclosing the tremendous impact that charge and orbital ordering have on the electric and magnetic properties of oxides [1] . In recent years, interfaces between different oxides, mainly AB O 3 perovskites, have been the backbone of an intensive research on emerging properties, such as highly conducting electron gases [2] , superconductivity [3] or polarization-dependent spin transfer [4] , paving the future of oxides towards oxide-based electronics. Electronic and structural reconstructions at interfaces among dissimilar oxides are driven primarily by electrostatic and strain-related effects. Moreover, interfaces have the genuine property of breaking the inversion symmetry of the system, thus promoting unique new properties such as engineered ferroelectric polarization and toroidal moments (see for instance Hwang et al. [5] ). These achievements have been made possible by the extraordinary progress in oxide thin-film growth, with atomic control of interfaces. However, it may be a surprise to realize that the free surface of thin-film oxides, being an example of the most dramatic interface, has received relatively little attention. Moreover, with Moore’s law as a driving force towards the integration of oxides in electronics, transition metal oxides are also being intensively investigated for green-energy applications, including catalysts for cost-effective electrochemical energy conversion processes of key relevance in water splitting, fuel cells and metal-air batteries. In this context, it has been recently shown that in transition metal oxides an archetypical example of a free-surface property such as the catalytic activity is intimately related to the number of electrons at 3 d -orbitals and the spin state [6] , [7] . This finding, while opening a way for a rational search for optimized catalysts, establishes a link between distinct views and approaches to materials science that may burst into renewed interest in electronic properties of free surfaces of oxides and faster progress in this field. In bulk cubic AB O 3 perovskites the octahedral coordination of cations at B -sites splits the 3 d -orbitals into a degenerated t 2 g triplet and a degenerated e g doublet with ( xy / yz / xz ) and ( x 2 -y 2 / 3z 2 -r 2 ) symmetries, respectively. Further lowering of the crystal-field symmetry breaks the degeneracy of x 2 -y 2 and 3z 2 -r 2 orbitals. A common driving force for such symmetry breaking is the half-filling of e g orbitals. In this situation, the strong electron-phonon coupling leads to a Jahn-Teller (JT) distortion of the B O 6 coordination polyhedron producing asymmetric B -O bonds that break the ( x 2 -y 2 / 3z 2 -r 2 ) degeneracy, thus modifying their electron occupancy and leading to complex orbital ordering ultimately responsible for the rich physics of many oxides [8] . Doubtlessly, because of the detailed understanding achieved on carrier filling and orbital effects in the colossal magnetoresistive oxides, this family of materials is the ideal candidate to explore the presumably subtle free-surface effects. In La 1-x Sr x MnO 3 , the electron occupancy in the ( x 2 -y 2 / 3z 2 -r 2 ) orbitals strongly depends on the hole doping level ( x ) and the strength of the JT distortion [1] . In bulk La 2/3 Sr 1/3 MnO 3 (LSMO), the partially filled ( x 2 -y 2 / 3z 2 -r 2 ) orbitals are responsible for the metallic character and the carrier-mediated Mn m+ –O −2 –Mn n+ double-exchange interaction is responsible for the ferromagnetic coupling. Epitaxial strain in LSMO thin films, similarly to the JT distortion, breaks the ( x 2 -y 2 / 3z 2 -r 2 ) degeneracy and dramatically changes their transport and magnetic properties [9] . In agreement with simple electrostatic expectations, it has been shown [10] , [11] , [12] , [13] that tensile strain favors x 2 -y 2 occupancy, whereas the compressive strain favors 3z 2 -r 2 occupancy, thus providing some understanding for the so-called magnetic and electric ‘dead’ layers [14] , [15] , observed in thin films. When two dissimilar oxides are brought together, charge transfer, electrostatic boundary conditions or/and elastic strain may also produce an additional modification of orbital filling, which can produce charge, orbital and spin reconstructions [16] , [17] . Similarly, interface-mediated bonding in heterostructures [18] , [19] largely depend on the relative position of the ( x 2 -y 2 / 3z 2 -r 2 ) orbitals at interfaces and thus their determination is of paramount importance. In this context, linear dichroism in the X-ray absorption (X-ray linear dichroism; XLD) is an extremely sensitive probe of the orbital occupancy of the distinct t 2 g - e g orbitals [20] , which has proven to be successful even at buried interfaces [21] . In LSMO thin films XLD has been used to firmly demonstrate that, while tensile strain favors the x 2 -y 2 occupancy, a compressive strain favors the 3z 2 -r 2 occupancy [11] , [12] , [13] . Here we explore the role of symmetry breaking at the free surface on the electron occupancy of e g orbitals in LSMO thin films. As the XLD sensitivity in total electron yield (TEY) decays exponentially within depths of the order of a few nanometres [22] , [23] our experiments have revealed the specific role of the free surface on the orbital occupancy of LSMO thin films. We will show that, although the ( x 2 -y 2 / 3z 2 -r 2 ) orbital configuration is primarily related to the strain state, an additional well-defined contribution emerges at the free surface, favoring the occupancy of out-of-plane e g orbitals. The final symmetry ( x 2 -y 2 or 3z 2 -r 2 ) depends on the surface atomic plane of LSMO which can be controlled by selecting the specific termination ((La,Sr)O or MnO 2 ) of the film. In agreement with theoretical predictions [16] , we will argue that the genuine contribution of the symmetry breaking at the free interface superimposes, and in some cases overrides, the strain-induced orbital occupancy, thus allowing the fine tailoring of the electron filling of surface ( x 2 -y 2 / 3z 2 -r 2 ) states and, concomitantly, their electric and magnetic properties. These results could pave the way for an active control of surface states and thereby surface functional properties of transition metal oxides. Sample fabrication and characterization We have used (001) LSMO epitaxial thin films with thicknesses ranging from ~1.5 nm (4 unit cells (u.c.)) up to ~60 nm (150 u.c.) grown on single crystalline SrTiO 3 (STO), LaGaO 3 (LGO), (LaAlO 3 ) 0.3 -(Sr 2 AlTaO 6 ) 0.7 (LSAT) and NdGaO 3 (NGO) substrates by RHEED (reflection high-energy electron diffraction) assisted pulsed laser deposition ( Supplementary Fig. S1 ). These substrates exhibit a mismatch (f=−0.3% for NGO, 0% for LSAT, 0.5% for LGO and 0.9% for STO) with respect to pseudocubic LSMO that allows changing the strain from compressive to tensile along the series. Two series of LSMO films have been grown. Relatively thick films, denoted NGO1, LSAT1 and LGO1 (≈150 u.c.) and STO1 (70 u.c.) were grown on the indicated substrates. A second series of ultrathin films were grown and are denoted as: NGO2, LSAT2 (4 u.c.) and STO2 (8 and 4 u.c.). (001)STO substrates with either mixed (SrO, TiO 2 ) terminations (as-received) or single terminated (either TiO 2 or SrO) were used (see Methods). (110)LSMO films on as-received (110)STO substrates were also grown. (001)LSMO films grown on either TiO 2 or SrO terminated (001)STO substrates display a morphology of terraces and steps ( Supplementary Fig. S2 ). The growth of these films was monitored by RHEED to ascertain a layer-by-layer growth and control the atomic termination ((LaSr)O or MnO 2 ) of the layer. The θ-2θ diffraction patterns around the (004) reflection of the thickest LSMO films (>70 u.c.) grown on different substrates are shown in Fig. 1a . Reciprocal interplanar distances 1/ d (004) ( d (004) is the interplanar (004) distance in LSMO) of all films have been normalized to that of the corresponding substrates (1/ d subs (004)) for better comparison of the strain state of the films. The shift towards a larger d subs (004)/ d (004) ratio (>1) for the STO1 film illustrates the substrate-induced in-plane tensile state and the resulting shrinking of d (004). The d subs (004)/ d (004) ratio is smaller for films grown on LGO1 as compared with STO1 and equals unity for LSAT1, as expected from the structural mismatch values. Similarly, the shift of d subs (004)/ d (004) to values <1 as observed for NGO1 illustrates the corresponding compressive in-plane strain. Reciprocal space maps confirmed that the in-plane cell parameters of LSMO match those of the corresponding substrates, thus indicating fully coherent growth. The observation of a fully strained state in the 150 and 70 u.c. films yields that the thinnest films used in this work (≈4–8 u.c.) are also fully strained. The Curie temperature T C and saturation magnetization M S for the thickest films ( Fig. 1b ) are similar to the corresponding bulk values (370 K, 590 emu cm −3 ); a depression of T C and M S is observed for the thinnest films ( T C <300 K, M S <400 emu cm −3 ) as typically found in ultrathin manganite films [11] , [12] , [15] , [24] . 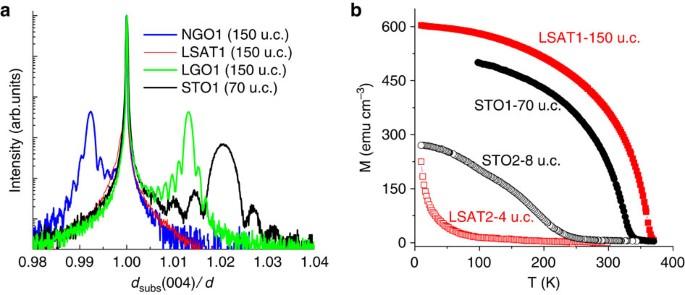Figure 1: Structural and magnetic characterization. (a) θ–2θ Scans for films grown on the indicated substrates: NdGaO3(NGO)-150 u.c., (LaAlO3)0.3-(Sr2AlTaO6)0.7(LSAT)-150 u.c., LaGaO3(LGO)-150 u.c. and SrTiO3(STO)-70 u.c.; (b) magnetization as a function of temperature for the Series 1 and Series 2 films grown on LSAT and STO substrates. Figure 1: Structural and magnetic characterization. ( a ) θ–2θ Scans for films grown on the indicated substrates: NdGaO 3 (NGO)-150 u.c., (LaAlO 3 ) 0.3 -(Sr 2 AlTaO 6 ) 0.7 (LSAT)-150 u.c., LaGaO 3 (LGO)-150 u.c. and SrTiO 3 (STO)-70 u.c. ; ( b ) magnetization as a function of temperature for the Series 1 and Series 2 films grown on LSAT and STO substrates. Full size image XLD on LSMO samples X-ray absorption spectroscopy (XAS) measurements were performed at the BACH beamline of the Elettra synchrotron radiation source, at the Mn L 2,3 -edges with photon polarization ( E ) parallel to the sample plane ( ) and almost perpendicular to it ( ) in total electron yield mode (see Methods). The XLD is calculated as the intensity difference ( − ) between the spectra measured with in-plane ( ) and out-of-plane ( ) polarizations. In (001)LSMO films, out-of-plane corresponds to E [001]; for in-plane , the polarization was chosen such as [100]. On (110)LSMO films, the out-of-plane direction corresponds to [110] and thus [110]; in-plane was obtained with E [001] ( Fig. 2a ). XLD gives information on the empty Mn-3 d states: larger (smaller) absorption for in-plane polarization indicates more in-plane (out-of-plane) empty states in the e g -band and thus a higher occupancy of out-of-plane (in-plane) orbitals [11] . In (001)LSMO films the out-of-plane direction is [001] ( c axis) and the in-plane is parallel to [100] and therefore and are proportional to the hole occupancies of 3z 2 -r 2 and x 2 -y 2 orbitals, respectively. Note that for (110)LSMO films, the out-of-plane direction is [110] and the [001] is in-plane and therefore and are proportional to the hole occupancies of x 2 -y 2 and of 3z 2 -r 2 orbitals, respectively ( Fig. 2a ). The XLD signals expected for unstrained as well as compressive and tensile strained films are shown by the simulated spectra in Fig. 2c . In Fig. 2b we have also depicted the effects of surface symmetry breaking inducing a preferential occupation of the orbitals oriented out-of-plane. 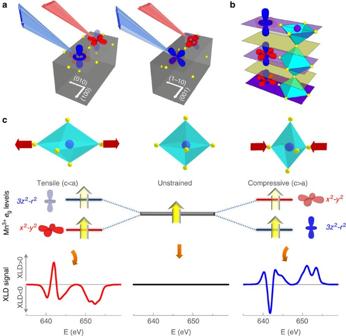Figure 2: Preferential orbital occupancy and linear dichroism. (a) Sketch of the polarized X-ray absorption measurements for both (001)- and (110)-oriented samples. In blue, incident radiation polarized out of the plane of the samples (); in red, incident radiation polarized in the plane of the samples (); (b) representation of the surface symmetry-breaking effects inducing a preferential occupation of the orbitals oriented out-of-plane. Purple layers account for MnO2planes while yellow layers account for (La,Sr)O planes; (c) top panel: representation of the MnO6octahedral distortions as a function of strain; middle panel: subsequent effect of the JT distortion on theeglevels of Mn3+ions; bottom panel: X-ray linear dichroism simulated for the Mn L-edge of Mn3+ion in a tetragonal crystal field withc<a(left), withc>a(right) and with octahedral field (centre)(see Methods). Figure 2: Preferential orbital occupancy and linear dichroism. ( a ) Sketch of the polarized X-ray absorption measurements for both (001)- and (110)-oriented samples. In blue, incident radiation polarized out of the plane of the samples ( ); in red, incident radiation polarized in the plane of the samples ( ); ( b ) representation of the surface symmetry-breaking effects inducing a preferential occupation of the orbitals oriented out-of-plane. Purple layers account for MnO 2 planes while yellow layers account for (La,Sr)O planes; ( c ) top panel: representation of the MnO 6 octahedral distortions as a function of strain; middle panel: subsequent effect of the JT distortion on the e g levels of Mn 3+ ions; bottom panel: X-ray linear dichroism simulated for the Mn L-edge of Mn 3+ ion in a tetragonal crystal field with c < a (left), with c > a (right) and with octahedral field (centre)(see Methods). Full size image We first discuss data collected for (001)LSMO films. Fig. 3 shows the XLD signal ( − ) derived from the normalized XAS spectra ( Supplementary Fig. S3 ), for the thicker (≥70 u.c.) films: NGO1, LSAT1, LGO1 and STO1. The dichroic signal around the high-energy L 2 absorption peak (648–660 eV) is the clearest indicator of the symmetry ( x 2 -y 2 / 3z 2 -r 2 ) of the occupied orbitals: a positive XLD signals 3z 2 -r 2 electron occupancy, whereas a negative XLD indicates x 2 -y 2 electron occupancy. Indeed, the simulated spectra included in Fig. 2c show that in this energy range, the XLD clearly changes its sign depending on the symmetry of the occupied states. Data in Fig. 3 display a clear trend: a positive XLD signal is observed for the NGO1 film, while a negative one is found for STO1. This indicates enhanced 3z 2 -r 2 electron occupancy for the compressively strained NGO1 film; conversely, the negative XLD signal for the tensile strained STO1 reflects a preferential x 2 -y 2 electron occupancy. These results are in agreement with previous findings [11] . However, a detailed inspection of the data for LGO1 and LSAT1 reveals an unexpected and remarkable 3z 2 -r 2 contribution, especially dramatic in LSAT1, where a clearly positive XLD is observed. We stress that the LSAT1 film is unstrained and thus a degenerated ( x 2 -y 2 / 3z 2 -r 2 ) occupancy should be expected and, accordingly, the XLD should vanish. 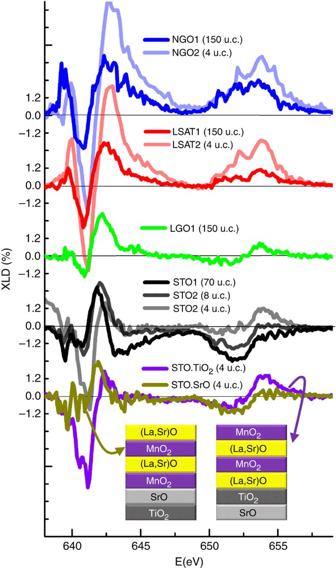Figure 3: X-ray linear dichroism. X-ray linear dichroism spectra of the Series 1 and Series 2 samples, including the films grown on single-terminated substrates (bottom spectra). Inset: sketches of the atomic planes in the single-terminated samples as induced by the SrTiO3substrate termination (SrO, left and TiO2, right). Figure 3: X-ray linear dichroism. X-ray linear dichroism spectra of the Series 1 and Series 2 samples, including the films grown on single-terminated substrates (bottom spectra). Inset: sketches of the atomic planes in the single-terminated samples as induced by the SrTiO 3 substrate termination (SrO, left and TiO 2 , right). Full size image Strain and surface effects on orbital occupation To quantify the orbital occupancy, the area under the L 2 peak in the XLD spectra (A XLD ) of Fig. 3 has been computed by integration in the photon energy range from 648 to 660 eV, as illustrated in Fig. 4 (bottom inset). The results are presented in Fig. 4 for the NGO1, LSAT1, LGO1 and STO1 films (solid squares). Expanding the integration range to the photon energy range between 638 and 660 eV to include energies around the L 3 peak leads to A XLD values that display the same trend ( Supplementary Fig. S4 ). The data clearly show that the strain is a driving force modulating the ( 3z 2 -r 2 / x 2 -y 2 ) occupancy ratio, as tensile strain promotes x 2 -y 2 occupancy, while compressive strain favors the 3z 2 -r 2 orbital filling. Moreover, the data in Fig. 4 lead to another important observation: strain alone cannot be the only driving force for the orbital energetic ordering. Note that the XLD spectra of the LSAT1 film ( Figs 3 and 4 )–which grows unstrained on the substrate ( Fig. 1 )–show a non-zero dichroism (A XLD (LSAT1)>0), which is at odds with what should be expected if strain was the only relevant factor. A natural origin for the observed positive XLD could be a vacuum-interface induced contribution to the orbital configuration, favoring occupancy of the out-of-plane 3z 2 -r 2 states. This assertion is corroborated by the inspection of the XLD spectra of the LGO1 film that, although having an intermediate tensile strain between LSAT1 and STO1, has a much reduced dichroic signal, close to zero (see Fig. 4 ). This result is expected from a positive contribution owing to the surface 3z 2 -r 2 orbitals counterbalancing the tensile favored x 2 -y 2 occupation. The free-surface contribution in Fig. 4 is visualized by the vertical upward shift of all the experimental XLD integrated data with respect to the origin (arrows in Fig. 4 ), thus indicating that a roughly constant 3z 2 -r 2 orbital occupation contribution adds in all XLD spectra, irrespectively of the strain state of the film. 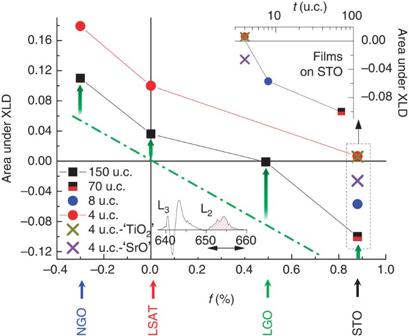Figure 4: XLD signal versus strain. Integrated area of the X-ray linear dichroism (XLD) signal as a function of lattice mismatch between La2/3Sr1/3MnO3and substrates. Negative values indicate preferential occupation of in-planex2-y2orbitals, while positive values indicate preferential occupation of3z2-r2orbitals. The dashed line is the expected variation of the integrated area due to strain effect; the arrows indicate the shift induced in the XLD spectra by the free-surface contribution. In the bottom inset the integration range (energy region of the L2peak) is indicated. Top inset: area under the XLD spectra as a function of thickness for samples grown on (001)SrTiO3substrates, including single terminated samples (crosses, as indicated in main panel legend). Figure 4: XLD signal versus strain. Integrated area of the X-ray linear dichroism (XLD) signal as a function of lattice mismatch between La 2/3 Sr 1/3 MnO 3 and substrates. Negative values indicate preferential occupation of in-plane x 2 -y 2 orbitals, while positive values indicate preferential occupation of 3z 2 -r 2 orbitals. The dashed line is the expected variation of the integrated area due to strain effect; the arrows indicate the shift induced in the XLD spectra by the free-surface contribution. In the bottom inset the integration range (energy region of the L 2 peak) is indicated. Top inset: area under the XLD spectra as a function of thickness for samples grown on (001)SrTiO 3 substrates, including single terminated samples (crosses, as indicated in main panel legend). Full size image The relevance of the free surface to the XLD with respect to other contributions, for example, the bulk of the film or even from the substrate/film interface can be probed by examining the XLD spectra of the thinnest films ( 8 u.c.). We note that the probing depth in TEY-XLD experiments is exponentially decaying within a few nanometers and, thus, we can check the surface vs. bulk contribution and/or the influence of the film/substrate interface. Accordingly, we measured the XLD spectra for the ultrathin NGO2, LSAT2 (4 u.c. ), STO2 (8 u.c.) and STO2 (4 u.c.) films ( Fig. 3 ). The calculated areas A XLD , obtained by integration of the XLD signal within the 648 to 660 eV photon energy range as above, are included in Fig. 4 (solid circles). It can be observed that, while A XLD on this set of data display the same dependence with strain than the thicker films (solid squares), the corresponding values display a shift towards more positive A XLD . The thickness dependence of the A XLD is explored in more detail for LSMO films grown on STO as shown in Fig.4 (top inset). Data indicates that the positive contribution to A XLD (that is, the 3z 2 -r 2 contribution) rises faster than exponentially when reducing LSMO thickness, thus signalling an enhanced contribution of 3z 2 -r 2 orbitals owing to the prevalence of the free-surface interface over the bulk of the film. These data indicate that Mn m+ ions at the free surface have a prominent 3z 2 -r 2 orbital occupancy. This conclusion is supported by the theoretical work of Calderon et al. [16] , who suggested that the free surface of (001)LSMO manganites should be prone to display a preferred occupancy of 3z 2 -r 2 orbitals due to the absence of apical oxygen coordination and the resulting reduction of the repulsive Mn-3 d ( 3z 2 -r 2 ) to O-2p(z) electron–electron interaction. It should be mentioned that the surface-related 3z 2 -r 2 contribution here disclosed is, in fact, a lower limit, as electron occupancy at 3z 2 -r 2 orbitals could have been partially reduced or screened by unavoidable surface contamination. Estimation of orbital polarization in bulk/surface of the films We have quantified the observed relative occupancy ( P ) of the 3z 2 -r 2 and x 2 -y 2 orbitals by taking into account the distinct contributions (orbitals at the free surface ( P s ) and at the bulk of the film ( P b )) depending on their position with respect to the surface and the attenuation depth ( δ ) of XAS (see Supplementary Methods ). It is found that the relative intensity of the dichroic signal, as inferred from data of Fig. 3 , when plotted as a function of the LSMO film thickness ( Fig. 5a ) can be well described (dashed lines) by a simple model (sketched in Fig. 5b ) that allows extracting the relative electron occupation at 3z 2 -r 2 and x 2 -y 2 orbitals of surface and bulk MnO 2 slabs ( P S and P b , respectively) and δ . From these fits (see Supplementary Methods for details) the surface electron occupancy in LSMO films is found to be of about ~75% at ( 3z 2 -r 2 ) and ~25% at ( x 2 -y 2 ) orbitals, thus clearly indicating a preferential 3z 2 -r 2 orbital filling; in contrast, the bulk contribution is found to depend on strain being about ~57.5%-( x 2 -y 2 ) in STO, 50%-( x 2 -y 2 ) in LSAT and ~46%-( x 2 -y 2 ) in NGO (see Supplementary Table 1 ). Therefore, bulk occupancy is determined by the epitaxial strain that, together with the genuine preferential surface 3z 2 -r 2 contribution, leads to the measured overall XLD signal. This quantitative analysis of data is in full agreement with the qualitative arguments presented above. The extracted probing depth ( δ ≈5 nm) is in good agreement with expectations [22] , [23] . 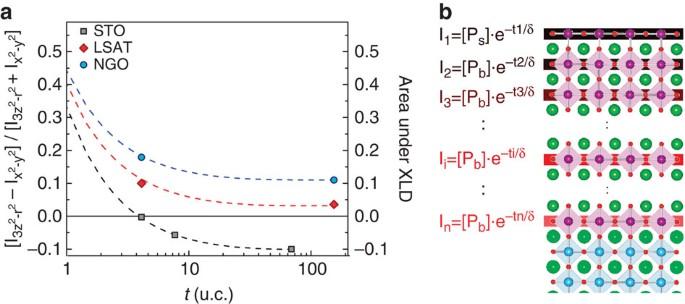Figure 5: XLD signal versus thickness of the samples. (a) Right axis (symbols): integrated area of the X-ray linear dichroism (XLD) signal of the samples grown on SrTiO3(001), (LaAlO3)0.3-(Sr2AlTaO6)0.7and NdGaO3substrates. Left axis (dashed lines): best fits of area under XLD signal to multilayer model as explained in the text. (b) Sketch of the model representing the contribution of the MnO2layers at a positionti(i=1…n, wheretnis the depth of the last layer of the film), having orbital occupancies P(3z2-r2)and P(x2-y2), to the measured intensity (Ii).PSandPbrepresent the difference of occupancies (P(3z2-r2)-P(x2-y2))at the surface (i=1) and at the bulk of the film (i>1). The exponential term reflects the attenuation (δ) of the outcoming signal. Figure 5: XLD signal versus thickness of the samples. ( a ) Right axis (symbols): integrated area of the X-ray linear dichroism (XLD) signal of the samples grown on SrTiO 3 (001), (LaAlO 3 ) 0.3 -(Sr 2 AlTaO 6 ) 0.7 and NdGaO 3 substrates. Left axis (dashed lines): best fits of area under XLD signal to multilayer model as explained in the text. ( b ) Sketch of the model representing the contribution of the MnO 2 layers at a position t i (i=1… n , where t n is the depth of the last layer of the film), having orbital occupancies P( 3z 2 -r 2 )and P( x 2 -y 2 ), to the measured intensity ( I i ). P S and P b represent the difference of occupancies (P( 3z 2 -r 2 )-P( x 2 -y 2 ))at the surface (i=1) and at the bulk of the film (i>1). The exponential term reflects the attenuation ( δ ) of the outcoming signal. Full size image In the data analysis shown in Figs 3 , 4 , 5 , the area under the XLD spectra of different films has been used to extract the relevant information on orbital occupancy. However, a detailed inspection of raw data in Fig. 3 shows that not only the total XLD area is changing but also fine details of spectra are gradually modified, when changing film thickness. This is particularly clear in the case of XLD data of LSMO films on STO where the spectra for LSMO films with different thicknesses are shown. The observed subtle variations reflect both the gradual change of the relative weight of the surface and bulk contributions to the XAS spectra and the corresponding crystal-field-determined electronic levels. Exponential decay determined by the probing depth δ calculated with the model described in the previous paragraph, in conjunction with parameters of the electronic structure of octahedrally and square-pyramidal oxygen coordinated Mn 3+ ions, have been used to simulate the XLD signal by means of atomic multiplet calculations [25] , leading to a reasonable reproduction of the thickness dependent spectra of films grown on STO (see Supplementary Methods for details and Supplementary Fig. S5 ). Tuning of orbital occupancy in single-terminated films A stringent test of the above conclusions can be obtained by comparing the XLD spectra of LSMO films with either MnO 2 or (La,Sr)O terminations at their free surface. In the MnO 2 terminated surfaces, the preferential 3z 2 -r 2 occupancy of Mn- e g orbitals is expected to be larger than in the (La,Sr)O terminated surfaces because of the square-pyramidal oxygen coordination of Mn m+ in the former and the octahedral oxygen coordination of the buried Mn m+ ions in the latter. This surface engineered terminations are achieved by the RHEED assisted layer-by-layer LSMO growth on (001)STO substrates having either TiO 2 or SrO terminations, respectively (see Methods), which promote either MnO- or (La,Sr)O- terminations, respectively. In Fig. 3 (bottom spectra) we include the XLD spectra of LSMO films, 4 u.c. thick, grown on TiO 2 or SrO terminated STO surfaces. Inspection shows that the LSMO/TiO 2 film displays a somewhat larger 3z 2 -r 2 than its LSMO/SrO counterpart. Integration of the XLD data as above allows evaluating the e g orbital occupancy; the corresponding A XLD values are included in Fig. 4 (crosses). The data clearly show that the A XLD (LSMO/SrO) value is significantly more negative than A XLD (LSMO/TiO 2 ), according to expectations. (110) oriented films It follows from the arguments presented above that the electron occupancy of out-of-plane orbitals is expected to be favored irrespectively of the particular crystallographic plane of LSMO considered. This has been assessed by comparing the XLD of LSMO films of similar thickness grown simultaneously on (001) and (110)STO substrates. In Fig. 6 we include data corresponding to films of 70 and 8 u.c. grown on (110)STO substrates. It can be observed that in the energy region as above (648 to 660 eV), the overall XLD of (110)LSMO films is mostly negative, implying that the out-of-plane absorption is larger than the in-plane , that is, A XLD ~( − ) <0. Importantly, the amplitude of A XLD is reduced when reducing film thickness thus indicating a gradual enhancement of the out-of-plane contribution when the surface contribution is larger. The A XLD values obtained by integration of the area under the XLD spectra are shown in Fig. 6 (inset). These data confirm that also for (110) LSMO films, the out-of-plane orbitals determine the electron orbital occupation at the surface. We stress that out-of-plane orbitals of free surfaces, that is, 3z 2 -r 2 for (001) and x 2 -y 2 for (110), largely contribute to the measured dichroism due to the low electron escape depth. 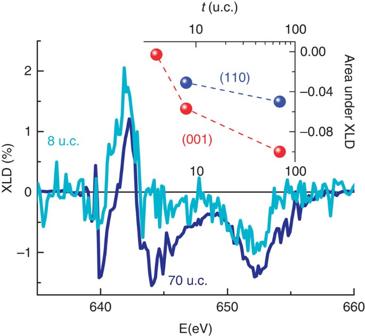Figure 6: (110) oriented samples. X-ray linear dichroism (XLD) signal of the samples grown on SrTiO3(110) substrates. Inset: area under XLD as a function of thickness for samples grown on (001) and (110) SrTiO3substrates. Figure 6: (110) oriented samples. X-ray linear dichroism (XLD) signal of the samples grown on SrTiO 3 (110) substrates. Inset: area under XLD as a function of thickness for samples grown on (001) and (110) SrTiO 3 substrates. Full size image We have provided experimental evidence that the symmetry breaking at the free interface of manganite thin films promotes a lifting of the degeneracy of the 3 d - e g electronic states of the transition metal and produces an enhanced electron occupancy of the out-of-plane orbitals, irrespective of their symmetry ( 3z 2 -r 2 or x 2 -y 2 ). The resulting orbital filling can be modulated through strain, to the point that the e g -band structure can be reversed for large enough tensile stress, populating preferentially the in-plane orbital states. Our data show that the ultimate orbital filling at the free surface of LSMO depends significantly on the stacking order of atomic planes, that is, -(La,Sr)O-MnO 2 or -MnO 2 -(La,Sr)O termination. The resulting surface electronic band structure should affect its physical properties, namely electric and magnetic, in a yet almost unexplored way; moreover, the surface chemistry of these films may be also largely modified. Interface properties such as wettability [26] , corrugation and hydrophobicity, or the catalytic activity are ultimately determined by the atomic/molecular structure of the surfaces. Although a few elegant experiments have been used to tailor the surface properties by external stimulus [27] , chemical reactions or changes in composition are most commonly used to modify surface properties. The present findings offer new prospects to dynamically adjust the surface-related reactivity by tuning the surface electron states via electric fields and strain. Recent progresses using voltage-controlled strain or orbital filling may be combined to reach active control of relevant surface electronic states. Samples LSMO epitaxial thin films with thicknesses ranging from ~1.5 nm (4 unit cells (u.c.)) up to ~60 nm (150 u.c.) have been grown by pulsed-laser deposition (PLD) using an excimer KrF laser. A high pressure RHEED (reflection high-energy electron diffraction) system was used to monitor growth characteristics and to determine the number of layers (u.c.) in layer-by-layer growth mode for the films grown on single-terminated STO. The deposition was made at an oxygen pressure of 0.2 mbar and keeping the substrate at a temperature of 725 °C. After growth, the films were allowed to cool down to room temperature. Single crystalline SrTiO 3 (STO), LaGaO 3 (LGO), (LaAlO 3 ) 0.3 -(Sr 2 AlTaO 6 ) 0.7 (LSAT) and NdGaO 3 (NGO) substrates were used. The film thickness has been determined either directly from RHEED images or X-ray reflectometry, or by controlling the number of PLD pulses after appropriate calibration of the growth rate (≈0.0155, nm per pulse). STO substrates with either mixed (SrO, TiO 2 ) terminations (as-received) or prepared to obtain a single termination (either TiO 2 or SrO) according common prescriptions [28] , [29] have been used. LSMO films of thickness (70 and 8 u.c.) were also grown on as-received (110)STO using identical growth conditions. Surface morphology Atomic force microscopy images were obtained in dynamic mode using an Agilent 5100 microscope. Digital images were analyzed using WSxM software. Structural and magnetic characterization High-resolution X-ray diffraction measurements (XRD) have been performed using a X’Pert diffractometer (Cu-Kα radiation). Magnetic properties were measured in a Quantum Design superconducting quantum interference device (SQUID) in the temperature range of 10–380 K with the magnetic field applied in the plane of the films along one of the main crystallographic directions. X-ray absorption XAS measurements were performed at the BACH beamline of the Elettra synchrotron radiation source. The spectra were measured at the Mn L-edge for the two polarizations (in-plane and out-of-plane) in a geometry such that the X rays impinge at grazing incidence onto the sample (60 degrees from the sample normal). The spectra were taken in TEY mode, measuring the photoelectron yield current produced at the sample surface with a picoammeter. The spectra normalization was made by dividing the spectra by a factor such that the L 3 pre-edge and L 2 post-edge have identical intensities for the two polarizations. After that, the pre-edge spectral region was set to zero and the peak at the L 3 edge was set to one. The spectra were recorded at temperatures well above the corresponding Curie temperatures (400 K for samples from Series 1 and 300 K for Series 2) to avoid any contribution from sample magnetic configuration to the XLD. Simulations Atomic model calculations were performed using CTM4XAS software using cubic crystal field 10 Dq=1.6 eV and adding a tetragonal distortion inducing a splitting of the t 2 g and e g levels equal to 3Ds−5Dt and 4Ds+5Dt, respectively. Here, we used Dt=0.02 and Ds=0.1 (for c>a) and Dt=−0.02 and Ds=−0.08 (for c<a) [25] . How to cite this article: Pesquera, D. et al. Surface symmetry-breaking and strain effects on orbital occupancy in transition metal perovskite epitaxial films. Nat. Commun. 3:1189 doi: 10.1038/ncomms2189 (2012).